Implementation of the CRISPR-Cas9 system in fission yeast Application of the CRISPR-Cas9 genome editing system in the model organism Schizosaccharomyces pombe has been hampered by the lack of constructs to express RNA of arbitrary sequence. Here we present expression constructs that use the promoter/leader RNA of K RNA ( rrk1 ) and a ribozyme to produce the targeting guide RNA. Together with constitutive expression of Cas9, this system achieves selection-free specific mutagenesis with efficiencies approaching 100%. The rrk1 CRISPR-Cas9 method enables rapid and efficient genome manipulation and unlocks the CRISPR toolset for use in fission yeast. The ‘Cas9’ Type II CRISPR-Cas system for genome editing has garnered considerable attention because of its high efficiency and flexibility. Originally discovered in prokaryotes, where it participates in genome defence against invading DNA, a minimal set of components has recently been defined and put to use in the specific editing of eukaryotic genomes [1] . This minimal system combines the RNase H/HNH-like endonuclease Cas9 and a single-guide RNA (sgRNA) containing both the trans-activating RNA and CRISPR RNA [2] . These components direct the cleavage of cognate DNA sequences determined by the sequence of the sgRNA, creating a double-strand break. The double-strand break will persist as long as the repair process that ensues is error-free resulting in the same target sequence, re-eliciting cleavage. Survivors of this cycle of cleavage and repair have acquired mutations in the target sequence that abrogate sgRNA/Cas9 recognition. The repair process can be directed to introduce specific changes by providing a DNA-editing template, containing the desired mutations, that engages in homologous recombination (HR) with the cleaved region. As unmutated sequences are repeatedly cleaved, leading to cell death, no additional markers are needed to select for mutation. Alternatively, this system can be used to tether protein factors to specific regions of the genome by their expression as chimeric fusion proteins with cleavage-deficient Cas9 mutants [3] , which retain their binding ability to sgRNA-programmable cognate sequences but do not cause mutagenic DNA damage. The CRISPR-Cas9 system has been adapted to virtually every model organism from baker’s yeast to mammals (reviewed in ref. 4 ). Expression of the sgRNA has unusual requirements because both its 5′ and 3′ ends need to be precisely defined in order to produce a functional Cas9/sgRNA ribonucleoprotein. This is usually achieved by means of the RNA Pol III promoter for the spliceosomal U6 snRNA that starts transcription in a defined G and terminates in a poly-T stretch. In yeast, this is not possible because the transcribed region contains cis -acting sequences integral to the promoter, preventing its use for expression of arbitrary sequences. This was circumvented in Saccharomyces cerevisiae through the use of a tRNA promoter [5] . In this system, a precursor with a leader RNA that is subsequently cleaved off at a precise location yields a mature sgRNA 5′ end, with the 3′ end defined by the RNA Pol III terminator. The fission yeast Schizosaccharomyces pombe has proven to be a useful model organism because of its higher degree of similarity to genomes of higher eukaryotes than the classic yeast model S. cerevisiae . S. pombe remains less well studied than S. cerevisiae , and lags behind in availability of molecular tools. In particular, lack of a portable RNA Pol III promoter to express sgRNA has prevented the implementation of the CRISPR-Cas9 system. Here we develop a CRISPR-Cas9 system that enables specific, precise and efficient genome editing in S. pombe . Its flexibility enables the use in fission yeast of the full range of CRISPR-derived tools for genome manipulation. sgRNA expression with the rrk1 promoter/leader RNA We sought to establish an sgRNA expression system in S. pombe . As, similar to those of S. cerevisiae , S. pombe RNA Pol III promoters include promoter elements in the transcribed region, we explored the possibility of using a transcript with a cleavable leader RNA. One such example is the rrk1 gene that codes for K RNA, a component of the RNAse P ribonucleoprotein [6] . Although its been reported that S. pombe rrk1 lacks a leader RNA, careful inspection of available high-throughput RNA sequencing data reveals that in mutants of rrp6 , a component of the exosome that degrades by-products of RNA maturation, rrk1 is preceded by a leader RNA of around 250 nucleotides [7] . We constructed an expression cassette by joining positions −1 to −358 of the rrk1 gene with the sgRNA sequence [5] , [8] , preceded by a CspCI restriction target site that serves as a placeholder for cloning of the targeting sequence ( Supplementary Fig. 1 ). As rrk1 is synthesized by RNA Pol II [6] , which has complex transcription terminators and yields polyadenylated transcripts, we cloned a Hammerhead Ribozyme [9] , [10] immediately downstream of the construct to precisely determine the 3′ end of the mature sgRNA ( Fig. 1a and Supplementary Fig. 1 ). Northern blotting and 5′ rapid amplification of cDNA ends (RACE) analysis revealed the accumulation of sgRNA with correct cleavage of the 5′ and 3′ ends, as well as the presence of a larger precursor ( Fig. 1b,c ). 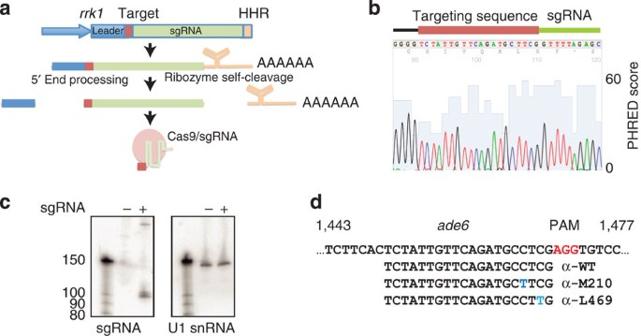Figure 1: sgRNA expression system. (a) Schema of sgRNA expression construct and processing. HHR: Hammerhead ribozyme. (b) 5′ RACE sequence. Only 4 bp of the oligodG attached to the 5′ end, resulting from the method, are shown. (c) Northern analysis of Cas9 expressing,ade6+strains with either no sgRNA vector or a sgRNA vector targeted againstade6-M210. Marker sizes are shown to the left and hybridization probe below. snRNA, small nuclear RNA. (d)ade6-targeting sequences. Figure 1: sgRNA expression system. ( a ) Schema of sgRNA expression construct and processing. HHR: Hammerhead ribozyme. ( b ) 5′ RACE sequence. Only 4 bp of the oligodG attached to the 5′ end, resulting from the method, are shown. ( c ) Northern analysis of Cas9 expressing, ade6+ strains with either no sgRNA vector or a sgRNA vector targeted against ade6-M210 . Marker sizes are shown to the left and hybridization probe below. snRNA, small nuclear RNA. ( d ) ade6 -targeting sequences. Full size image Mutagenesis of ade6 As a proof of principle of the CRISPR-Cas9 mutagenesis system, we attempted the editing of the ade6 gene, which when mutated causes accumulation of a red coloured precursor in media with low adenine [11] . We generated sgRNA constructs targeting three different alleles of ade6 : ade6+ ( WT ), ade6-M210 and ade6-L469 . The M210 and L469 mutations are located within a 3-bp window near a protospacer adjacent motif necessary for Cas9/sgRNA recognition ( Fig. 1d ), and are easily characterized because they yield deep red colonies and cause an Xho I restriction site polymorphism. As a DNA template for directed HR, we generated PCR products containing the WT and M210 alleles, as well as a non-homologous amplicon of the same size as control. We transformed strains containing wild type (WT), ade6-M210 , ade6-L469 or ade6-M216 (an allele mutated outside of the targeted region yielding light pink colonies) alleles with an adh1 :Cas9 constitutive expression construct and rechecked the ade6 phenotype of the transformants to ensure that Cas9 induces no changes without the sgRNA. We then picked individual transformants from each strain, transformed them with all combinations of one sgRNA expression construct and one mutation donor DNA, and spread them onto Edinburgh Minimal Media supplemented with a low concentration of adenine. We scored the phenotype of the colonies generated, and picked individual colonies for sequencing of the ade6 gene. Transformation of sgRNA targeting alleles different from the one present in the transformed strain yielded no changes in phenotype. This indicates that the single-nucleotide polymorphisms were sufficient to confer complete specificity to the mutagenesis ( Supplementary Fig. 2 ). When transformed with a sgRNA targeting the allele present in the strain, the Cas9-expressing transformants exhibited a wide variation of mutagenesis efficiencies. Some of them (8 out of 12) changed colour (white to red, red to white and pink to red) with efficiencies between 50 and 98%, with the highest efficiencies corresponding to those co-transformed with an HR template donor that changes the targeted sequence (85–98%, Supplementary Fig. 2 ). Targeting of the WT sequence present in the WT and M216 strains (yielding white and pink colonies, respectively) resulted in the generation of dark red colonies, indicating that the targeted region acquired new mutations that phenocopied the M210 and L469 mutations. Conversely, targeting of the ade6-M210 and ade6-L469 alleles resulted in the appearance of white colonies indicating reversion to the WT allele. However, a portion of the Cas9-expressing transformants (4 out of 12) were resistant to CRISPR-mediated mutagenesis, with mutation efficiencies between 0 and 5% even when the allele present was targeted by the sgRNA. We sequenced the ade6 gene from unmutated and mutated colonies (according to their colour) in experiments from mutagenesis-competent transformants ( Supplementary Fig. 3 ). The sequencing results show that when the allele present in the strain is targeted by the sgRNA, mutagenesis occurs through two different mechanisms depending on the HR donor template co-transformed. If the donor template is homologous to the targeted region and it provides a mutation that would confer resistance to cleavage by the Cas9/sgRNA, almost all the mutated colonies had acquired the template mutation (22/23), indicating that repair of the cleavage had occurred through HR with the donor template. However, when the donor template encodes the same allele that is being targeted in the strain or is non-homologous to the targeted region (control), the resulting mutations were small deletions and insertions at the cleavage point, typical of repair through non-homologous end joining. Colonies that retained the original phenotype also showed the original genotype in their sequence, indicating that they had somehow become resistant to Cas9/sgRNA cleavage without mutating the targeted sequence. If the sgRNA transformed targeted a different ade6 allele from that present in the strain, no mutations were detected. The transformation efficiencies observed in the mutagenesis-competent clones differed depending on the sgRNA used: they were very high (10 4 c.f.u. per μg) if it targeted an allele different from the one present in the strain, but dropped (to between 10 and 10 2 c.f.u. per μg) when the sgRNA targeted the allele present in the strain. This suggests that the combination of Cas9 with a targeting sgRNA challenges the survival of the transformant. In contrast, Cas9-expressing transformants resistant to CRIPSR mutagenesis showed consistently high transformation efficiencies, independently of the sgRNA used, indicating that cleavage of the target was impaired in these clones. Toxicity of Cas9 leads to inactivating mutations We sought to investigate the source of the drastic differences in CRISPR competency of the different Cas9-expressing clones. We hypothesized that mutations or rearrangements in the Cas9- and/or sgRNA-expressing plasmids could render them inactive. To test this hypothesis, we recovered the transformed plasmids from CRISPR-competent and -incompetent clones, and characterized them by restriction digest and sequencing. Both sgRNA- and Cas9-expressing plasmids were intact in CRISPR-competent clones (not shown). sgRNA plasmids from CRISPR-incompetent clones were also intact. In contrast, Cas9-expressing plasmids from CRISPR-incompetent clones exhibited rearrangements and mutations that would render them inactive ( Supplementary Fig. 4 ). The relatively high frequency of these events suggested that Cas9 inactivation underwent positive selection, implying that Cas9 overexpression is toxic to fission yeast, even without a sgRNA. Stochastic mutations of Cas9 would overcome the chosen transformant resulting in sporadic loss of CRISPR competency. We tested this hypothesis generating a construct that expresses Cas9 driven by the inducible nmt1 promoter, which is active in the absence of thiamine. The size of the colonies transformed with this construct depended on the induction conditions: plating onto media without thiamine (nmt1 promoter active) resulted in colonies much smaller than those plated in media with thiamine (nmt1 repressed) indicating impaired growth upon Cas9 expression ( Supplementary Fig. 5 ). Accordingly, clones obtained from the nmt1-repressed plate showed a drastically reduced growth rate when grown in liquid media without thiamine ( Supplementary Fig. 5 ). We conclude that Cas9 overexpression is toxic to fission yeast, and that maintenance of Cas9-expressing clones carries the risk of incapacitating mutations that impede CRISPR genome editing. A combined expression vector overcomes Cas9 inactivation In order to prevent the selection of Cas9 mutations in the mutagenesis protocol, we evaluated the efficiency of mutagenesis induced by a combined vector expressing both Cas9 and the sgRNA. This approach has the added advantage of requiring a single transformation instead of two. We cloned the adh1 promoter-driven Cas9 expression cassette into the sgRNA expression plasmid, and then cloned the ade6+ -, ade6-M210 - and ade6-L469 -targeting sequences into the sgRNA cassette. We then transformed them into the same ade6+ , ade6-M216 , ade6-M210 and ade6-L469 strains used in the two-plasmid system, along with the same ade6+ , ade6-M210 and control HR donor templates, in all combinations. The results are summarized in Fig. 2 . Transformation of the single-plasmid vector with a sgRNA targeting the allele of ade6 present in the strain caused a high frequency of mutation with robust reproducibility. Recapitulating the results observed in the CRISPR-competent Cas9-expressing clones, the highest efficiencies (85–90%) were obtained by co-transformation with an HR template that mutates the targeting sequence. 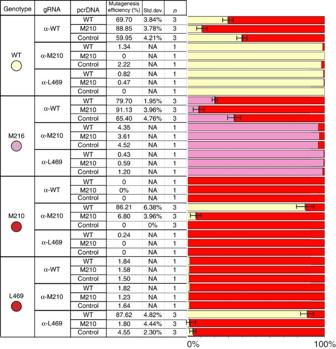Figure 2:ade6mutagenesis. The original genotype and phenotype are shown in the first column, the sgRNA expression vector in the second, the PCR product used as HR template in the third, followed by average mutation efficiency, standard deviation and number of experiments. The phenotype of the survivor colonies is shown in stacked bar format, with error bars depicting standard deviation. NA, not applicable. gRNA, single guide RNA; pcrDNA, HR donor template. Figure 2: ade6 mutagenesis. The original genotype and phenotype are shown in the first column, the sgRNA expression vector in the second, the PCR product used as HR template in the third, followed by average mutation efficiency, standard deviation and number of experiments. The phenotype of the survivor colonies is shown in stacked bar format, with error bars depicting standard deviation. NA, not applicable. gRNA, single guide RNA; pcrDNA, HR donor template. Full size image Epitope tagging by CRISPR-Cas9 editing We then attempted a real-life application of CRISPR mutagenesis by inserting an N-terminal epitope tag into cdc6 , the catalytic subunit of DNA polymerase Delta. N-terminal tagging by classic means involves a multistep process with antibiotic markers and the generation of large transforming fragments. We created an sgRNA targeting the N-terminus of cdc6 , and generated a PCR product containing a 3xHA tag in frame with the N-terminus of cdc6 , destroying the targeted site, with 200 bp homology regions on both sides of the tag ( Supplementary Fig. 6 ). We co-transformed these constructs into a WT strain, and picked five clones at random for characterization of cdc6 . All five clones showed the expected size increase by PCR, and western blotting confirmed that a protein of size corresponding to that of Cdc6 tagged with 3xHA was expressed ( Supplementary Fig. 6 ). S. pombe is the model organism of choice for studies of chromosome biology, because of its conservation of crucial aspects of chromosome function, such as complex heterochromatic centromeres, with higher organisms. However, modification of the S. pombe genome is often laborious, time consuming, and requires the use of marker genes that may interfere with the phenomenon being investigated. Delitto perfetto approaches that subsequently remove the marker genes require multiple selection steps and screening of large number of candidate colonies to obtain the desired modification [12] . Furthermore, owing to the lower efficiency of HR with exogenous DNA observed in S. pombe as compared with S. cerevisiae , extended homology regions are required, necessitating additional cloning steps [13] , [14] . As targeted cleavage of the unmutated sequence constitutes a built-in negative selection, CRISPR-Cas9 mutagenesis achieves near complete efficiencies and obviates the need for selectable markers. The single vector expressing Cas9 and the sgRNA is marked with ura4 , allowing for plasmid removal by counterselection with 5-fluoroorotic acid to enable subsequent mutagenesis of additional targets. We expect that the flexibility of the rrk1 sgRNA expression system will allow for implementation of the full Cas9 toolset, from Cas9/sgRNA systems with alternate protospacer adjacent motifs [15] to nicking and catalytic dead mutants of Cas9 (refs 3 , 16 ). The RNA Pol II-expressed rrk1 /Hammerhead ribozyme cassette may also prove useful in other situations where expression of RNA of defined arbitrary length and sequence such as short interfering or long non-coding RNA (lncRNA) is needed, an advantage over RNA Pol III systems. The methods and reagents presented here will prove useful for genomics research in S. pombe by enabling rapid and specific genome editing. Constructs All oligonucleotides are described in Supplementary Table 1 . All plasmids ( Supplementary Table 2 ) are available from the Addgene repository (http:// www.addgene.org ). Cas9 was built by Gibson assembly [17] of two Cas9 fragments amplified from plasmid p414-TEF1p-Cas9-CYC1t (Addgene; Oligos OM446/OM449 and OM447/OM448), introducing a silent mutation in the CspCI site, into plasmid pART1 digested with Pst I, resulting in plasmid pMZ222. The sgRNA expression construct was built by Gibson assembly of a synthetic double-stranded DNA containing the rrk1 promoter and leader RNA, the CspCI placeholder and the sgRNA ( Supplementary Fig. 1 ), into plasmid pUR19 (OM473/OM474), yielding pMZ252. We inserted the Hammerhead ribozyme from the satellite RNA of Tobacco Ringspot Virus (OM552/OM553) immediately downstream of the sgRNA by Gibson assembly with plasmid pMZ252 (PCR-amplified with OM550/OM551), yielding pMZ283. The ade6 -targeting sgRNA constructs were built by digestion of pMZ283 with CspCI and ligation with double-stranded oligonucleotides with the desired sequence (oligonucleotides OM450/OM456 (WT); OM452/OM457 (M210); OM454/OM458 (L469)) yielding pMZ284 (wt), pMZ285 (M210) and pMZ286 (L469). The combination Cas9/sgRNA plasmid pMZ374 was cloned by amplifying the adh1:Cas9 expression cassette (oligonucleotides OM554/OM555) and inserting it into the ZraI site of pMZ283 by Gibson assembly. Targeting sgRNA were cloned into the CspCI placeholder as with pMZ284-6. The nmt1:Cas9 construct was made by Gibson assembly of a Cas9 fragment (OM777/OM778), the nmt1 promoter (OM801/OM802) and the Bam HI/ Sph I-digested pART1 vector, resulting in vector pMZ373. The cdc6-Nterm-targeting sgRNA was made cloning oligos OM817/OM818 into pMZ283. The DNA provided as an HR donor template was produced by PCR of the targeted region in the case of WT and M210 (OM12/OM13), or an unrelated PCR product contained within the reb1 gene as control (OM100/OM101). PCR products were purified with silica membrane columns (Epoch Life Science) and used directly for transformation. To create the haemagglutinin (HA)-tagging template, HA was amplified from pFA6-3xHA (OM821/OM822). The 5′ and 3′ regions flanking the cdc6 start codon were amplified with OM820/OM823 and oM825/oM824, respectively. These three fragments were then gel purified and joined by cross-over PCR with (OM820/OM825). Transformation and mutagenesis experiments All strains used contained the ura4-D18 and leu1-32 alleles, and one of four ade6 alleles (WT, M210, L469 or M216). Strains were grown in 5 ml of MB media (Sunrise Science, Products #2016) with the appropriate supplements at 32 °C to mid-log phase (OD=0.5) and transformed by the Lithium Acetate/PEG/Heat-shock method [18] . Transformation of pMZ222 was selected on Dropout media without Leucine. All mutagenesis experiments were carried out by cotransformation of 1 μg of the sgRNA construct (for Cas9 expressing strains) or Cas9/sgRNA construct (for single-step mutagenesis), and 1 μg of the PCR product used as HR template. 5 ml of mid-log phase cultures were grown in MB media (Sunrise Bioscience #2016) with supplements, transformed as above, spread onto Edinburgh Minimal Media (EMM, US Biological, #E2205) plates supplemented with 10 mg l −1 adenine immediately after heat shock and grown at 32° C for 4 days. For colony, PCR individual colonies were picked, restruck to single colonies, boiled in 0.02 M NaOH for 10 min, and the ade6 -targeted region was PCR amplified and sequenced. 5′ RACE analysis WT strains expressing Cas9 via vector pMZ222, transformed with a sgRNA directed against the ade6-M210 allele were picked form single colonies and grown in EMM media to mid-log phase and harvested and total RNA was extracted with the hot phenol method. 5 μg of total RNA was used with the 5′ RACE System Version 2.0 kit (Life technologies) using OM546 for reverse transcription and OM547 for nested PCR, cloned by TopoTA (Life Technologies) and sequenced. Northern blotting analysis WT strains expressing Cas9 via vector pMZ222, either without sgRNA vector or transformed with a sgRNA directed against the ade6-M210 allele (to avoid any selection effects from the targeting and cleavage of the endogenous allele), were picked from single colonies, grown in EMM media to mid-log phase, harvested and total RNA was extracted with the hot phenol method. 5 μg of total RNA was run alongside a radioactively labelled Decade Marker (Life Technologies) on a 8% polyacrylamide gel electrophoresis (PAGE) with 8 M urea and blotted onto charged nylon membrane by semi-dry transfer. The blot was hybridized to labelled oligonucleotides OM599 (U1) or OM 546 (sgRNA). Growth rate measurements Colonies transformed with pMZ373 were plated in EMM plates with the appropriate supplements and either with or without 10 μM thiamine, grown for 4 days and photographed. Six colonies from the plate with thiamine were picked and used to seed cultures of 200 μl EMM with supplements (three with and three without 10 μM thiamine) at equivalent initial OD in a BioTek ELx808IU absorbance microplate reader set incubate at 32 °C and to shake the culture and take an OD reading every 30 min. HA-tag characterization A ura4-D18, leu1-32 strain was mutagenized as described above, offering the HA-tagged cdc6 N-terminus fragment as HR donor template, and plated onto media selective for the Cas9/sgRNA vector. Five colonies were picked at random and colony PCR performed as above. The same colonies were grown in EMM with the appropriate supplements to mid-log phase, pelleted and boiled in Laemmli loading buffer, run in an 10% SDS–PAGE gel and transferred by semi-dry transfer in 1 × Bjerrun transfer buffer onto 0.2 μm pore nitrocellulose. The membrane was blocked with 5% non-fat milk in 1 × Tris-buffered saline-tween and incubated with anti-HA antibody (Abgent, AP1012a) or with anti-Sap1 antibody [18] diluted 1:1,000 in blocking buffer, then developed with secondary anti-rabbit-HRP conjugate and ECL (GE). How to cite this article : Jacobs, J. Z. et al . Implementation of the CRISPR-Cas9 system in fission yeast. Nat. Commun. 5:5344 doi: 10.1038/ncomms6344 (2014).